Hydrolase–like catalysis and structural resolution of natural products by a metal–organic framework The exact chemical structure of non–crystallising natural products is still one of the main challenges in Natural Sciences. Despite tremendous advances in total synthesis, the absolute structural determination of a myriad of natural products with very sensitive chemical functionalities remains undone. Here, we show that a metal–organic framework (MOF) with alcohol–containing arms and adsorbed water, enables selective hydrolysis of glycosyl bonds, supramolecular order with the so–formed chiral fragments and absolute determination of the organic structure by single–crystal X–ray crystallography in a single operation. This combined strategy based on a biomimetic, cheap, robust and multigram available solid catalyst opens the door to determine the absolute configuration of ketal compounds regardless degradation sensitiveness, and also to design extremely–mild metal–free solid–catalysed processes without formal acid protons. The absolute structural configuration of natural products has been historically verified by total synthesis [1] , either from commercial compounds or, more conveniently, from fragments of the compound after controlled degradation and re-synthesis. However, the later approach is often hampered by the sensitiveness of natural complex molecules. For instance, the glycosyl bond [1] (–O–CR 2 –O–) is prevalent in natural products since glycosidase (hydrolase) enzymes are widespread in all domains of life to generate (and break) ketals with an extremely high selectivity, at neutral pH in water, by the combined action of some amino acid residues in the confined enzyme electrostatic pocket. However, classical synthetic chemistry operates under much harder conditions, by using formal acids (i.e., protons and Lewis metal cations) or bases (i.e., inorganic bases and amines), which are clearly incompatible with the outstanding structural richness and sensitive functionality of ketals in Nature, and severely hampers the absolute determination of natural product structures by simple chemical degradation [2] , [3] . Microporous solids may mimic enzymes with their active catalytic species in an electrostatic confined space [4] , [5] . Indeed, simple microporous aluminosilicates are good catalysts for ketal deprotection [6] , but they show low selectivity towards other acid sensitive functional groups, since the catalytic activity comes from acid protons associated with the solid network [7] . Early observations in microporous pure silicates showed that densely packed and interacting Si–OH groups, called silanol nests, naturally generate an acid site for catalysis without the participation of a formal proton [8] , [9] , however, the concept could not be extended to the organic functionalities present in enzymes, such as alcohols, since alcohols tend to generate either alkoxides [4] or carbocationic species [10] rather than acid sites, unless water [11] or acetic acid [12] are co-added. These precedents severely preclude simple alumisolicates to be used as catalase-like catalysts [13] with extremely mild, bifunctional acid/base sites. Metal–organic frameworks (MOFs) [14] are porous crystalline materials amenable to single-crystal X-ray crystallography [15] (SCXRD), with a great synthetic control of their high-dimensional architectures and concomitant porosity by a fine tuning of the functionalities decorating their channels using both pre- or post-synthetic [16] , [17] methods. Indeed, their thrilling host–guest chemistry has led to the selective incorporation of gases, solvents, small molecules or more complex molecular systems [18] , [19] . Besides, advances like the crystalline sponge method [20] , developed by Fujita’s group, allows the absolute determination of organic molecules within the MOF framework [21] , [22] , [23] . Thus, seems plausible to go one-step further for the development of novel families of MOFs, specifically designed to combine the catalytic in-situ formation [1] , [24] , [25] , [26] , [27] , [28] , capture [29] , [30] , [31] , organization [19] , [32] and retention of very sensitive unknown organic species within their functional channels [33] . Herein, we report that a previously reported [30] , [31] , [34] highly robust crystalline MOF-derived from the natural amino acid l -serine and whose micropores are densely decorated with methyl alcohol groups is capable to accommodate relatively big natural products, and performs, in a single operation, ketal deprotection and structural determination of sugars [1] and flavonoids of known and unknown absolute configuration. After selectively incorporating, untouched, the fragment of unknown chirality into the MOF, the solid structure is resolved by SCXRD to give the absolute configuration of the adsorbed organic fragment (Fig. 1a ) and, thus, of the natural product. Fig. 1: MOF-catalyzed selective hydrolysis of glycosyl bonds of sucrose 1. a Schematic representation of the one-pot selective hydrolysis/adsorption/crystal resolution of a natural product within a MOF. b 1 H NMR spectra of sucrose 1 before and after selective hydrolysis with MOF 2 , and SCXRD resolution of fructose fragment 1a . c Evolution with time of naringin 10 in CD 3 CN after reaction with MOF 2 at 60 °C, followed by 1 H NMR. d Hydrolysis and incorporation of the alkyl part of naringin 10 into MOF 2 or MOF 3 with time for different amounts of MOFs (left) and initial rate as a function of the amount of MOF 2 employed (right), according to 1 H NMR integrations. Reaction rates were measured with the initial points up to 30% conversion. Lines are a guide to the eye. Error bars account for a 5% uncertainty. Full size image 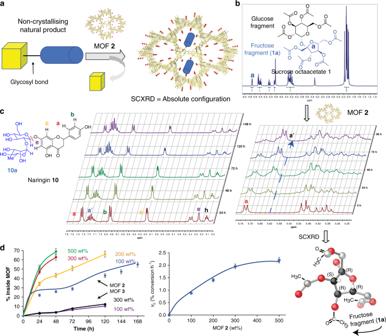Fig. 1: MOF-catalyzed selective hydrolysis of glycosyl bonds of sucrose 1. aSchematic representation of the one-pot selective hydrolysis/adsorption/crystal resolution of a natural product within a MOF.b1H NMR spectra of sucrose1before and after selective hydrolysis with MOF2, and SCXRD resolution of fructose fragment1a.cEvolution with time of naringin10in CD3CN after reaction with MOF2at 60 °C, followed by1H NMR.dHydrolysis and incorporation of the alkyl part of naringin10into MOF2or MOF3with time for different amounts of MOFs (left) and initial rate as a function of the amount of MOF2employed (right), according to1H NMR integrations. Reaction rates were measured with the initial points up to 30% conversion. Lines are a guide to the eye. Error bars account for a 5% uncertainty. Glycolysis of natural products of known structure Figure 1b shows the proton nuclear magnetic resonance spectra ( 1 H NMR) of a solution of sucrose octaacetate 1 (neat sucrose was not soluble under reaction conditions) recorded with time in the presence of the amino acid-based catalytic MOF 2 , which features hexagonal pores densely decorated with –OH groups, and with formula {Ca II Cu II 6 [( S,S )-serimox] 3 (OH) 2 (H 2 O)}. 39H 2 O ( 2 ) (where serimox [30] , [31] , [34] = bis[( S )-serine]oxalyl diamide, see also Supplementary Fig. 1 ). Isostructural MOF alamox ( 3 ) of formula {Ca II Cu II 6 [( S,S )-alamox] 3 (OH) 2 (H 2 O)}. 32H 2 O (where alamox = bis[( S )-alanine]oxalyl diamide) without alcohol but only methyl pending groups was used for comparison. The results show that the NMR signal corresponding to the ketal linkage (a) and, in general, all the signals associated with one of the parts of ketal 1 , the fructose fragment 1a , progressively disappears in solution in the presence of MOF 2 , while the glucose fragment 1b remains. Conversely, no hydrolysis was observed with MOF 3 , lacking confined alcohol groups. Gas chromatography coupled to mass spectrometry (GC-MS) analyses confirmed the nearly exclusive presence of glucose fragments 1b in solution after treatment with MOF 2 (Supplementary Fig. 2 ). SCXRD of a crystalline sample of MOF 2 reacted with 1 (see “Methods” and Supplementary Methods ) rendered a new host–guest material with formula ( 1a )@{Ca II Cu II 6 [( S,S )-serimox] 3 (OH) 2 (H 2 O)}. 19H 2 O ( 1a@2 ) (where 1a = 1,3,4,6-Tetra- O -acetylfructofuranoside), whose crystal structure as well as absolute configuration could be elucidated by SCXRD analysis (see Fig. 2 and Supplementary Table 1 and also an in-depth analysis of 1a@2 crystal structure in Supplementary Methods ). The results show that the only fragment found inside MOF 2 is fructose 1a and not any glucose derivative (Fig. 1b and Supplementary Figs. 3 – 6 and Fig. 2 and crystallographic section in SI for details). These fragments, well defined by furanose ring, that is completely assigned by electron density maps, reside in the pores of MOF 2 anchored by means of strong hydrogen bonds involving locked water molecules, which act as a bridge between serine moieties and fructose molecules. So, the alcohol groups show a prominent role, providing the suitable polar environment to host fructose molecules, effectively retained and organized within the pores. Fig. 2: Crystal structure of 1a@2. a Perspective view along c crystallographic axis of a single channel underlining pores filled by guest molecules depicted as blue sticks with the only exception of oxygen atoms, depicted as red spheres. The H-bond interactions are depicted as red dashed lines. Disordered positions of lattice water molecules having a key role in host–guest interactions are highlighted (see details of refinement in Supplementary Methods ). b Supramolecular chains of 1a molecules packed in pores of 2 propagating along the direction of channels (all possible orientations are included). Carbon are represented by blue sticks whereas oxygen atoms of guest molecules and water molecules mediating host–guest interactions are represented by red spheres. Full size image In order to better visualize and also to determine the relative catalytic hydrolysis rate compared to alcohol dihydroxylation (a representative competitive reaction in natural product degradation), the benzaldehyde and cyclohexanone ketals 4 and 5 , and 2-phenyl-2-propanol 6 , were employed as substrates for ketal hydrolysis and the dehydroxylation reaction, respectively (Supplementary Fig. 7 ). The kinetic results showed the formation of carbonyl compounds 7 and 8 at a significant rate for MOF 2 (5 mol% of MOF structural units respect to the substrate), but not for MOF 3 . Remarkably, despite the formation of alkene 9 may be expected to be extremely easy with a highly stable benzylic carbocation intermediate, the hydrolysis rate is twice for the dehydroxylation of 6 . These results confirm that MOF 2 selectively catalyzes the hydrolysis of glycosyl bonds without significant degradation of alcohol-substituted chiral carbons. To further validate the extremely mild solid-catalyzed glycosyl bond-breaking reaction, the commercially available flavonoid naringin 10 (Supplementary Fig. 8 ), with a more complex glycosyl structure, was treated with catalytic amounts of MOFs 2 and 3 . Figure 1c shows the progressive disappearance of the 1 H NMR signals corresponding to the alkyl fragment 10a respect to the aromatic part, the latter evolving to a different product in solution which, according to NMR and GC-MS, may be assigned to the oxidized quinone derivative. The spontaneous oxidation of the aromatic part in flavonoids, after losing the stabilizing glycosyl fragment, was expected according to the literature [10] , [35] . Figure 1d shows the increase in the hydrolysis rate of naringin 10 with MOF 2 , but not with MOF 3 , the latter in the same range that the hydrolysis rate without catalyst. All the results above, together, strongly support that MOF 2 selectively breaks glycosyl bonds in natural products and, concomitantly, adsorbs the so-formed alkyl chains, such as 1a in sucrose and 10a in naringin. Glycolysis and structural resolution of Brutieridin 11 Aiming to further test our hypothesis, we studied a unique class of flavonoids that is found in bergamot fruit (Citrus Bergamia Risso et Poiteau) which, in addition to other citrus species such as naringin 10 , neohesperidin and neoeriocitrin, contains a relevant concentration of the anti-cholesterol agent 6- O- hydroxymethylglutaryl (HMG) ester derivative brutieridin 11 (Fig. 3a and Supplementary Figs. 9 and 10 ) [36] , [37] , [38] , [39] . Flavonoids are secondary metabolites widespread in Nature and involved in different metabolic processes, offering potential clinical alternatives to current treatments. However, so far, the challenging characterization of this kind of flavonoids has been carried out by the combination of High-performance liquid chromatography, MS, and NMR techniques, which have severe shortcomings for the proper identification of their chiral centers. For instance, brutieridin 11 has been isolated and identified with the formula hesperetin 7-(2′′-R-rhamnosyl-6′′-(3′′′′-hydroxy-3′′′′-methylglutaryl)-glucoside [36] , but all attempts to crystallize it, thus determining its crystal structure and unveiling its chiral nature, have been unsuccessful so far. Brutieridin 11 presents two glycosidic bonds and, beyond other sensitive functionalities, several secondary and tertiary chiral alcohols along its chemical structure. It is noteworthy the presence of an alcohol group flanked by two different carboxylic groups in beta position (fragment 11a , Fig. 3a ), an extremely sensitive chemical aggrupation prone to suffer degradation under both acid or basic conditions, since the tertiary alcohol dehydrates under acid conditions to generate a stable alkene conjugated to any of both carboxylic groups or, conversely, the alpha carbon to the carboxylic groups deprotonates under basic conditions to generate the same degraded products. These easy acid or base-triggered reactions, together with the interferences and potential side reactions caused by the phenol, ester, ketone and ether groups also present in brutieridin 11 , makes extremely difficult the selective degradation of this natural product by any classical deketalization method. Fig. 3: Hydrolysis of brutieridin 11. a Chemical structure of brutieridin 11 . Gray-colored ellipse highlights the fragment 11a , which contains the chiral carbon and encapsulates within the MOF after the break of the glycosidic bonds. b Chemical structure and 13 C NMR spectrum of 11- 13 C in solution (black line), and MAS solid 13 C NMR spectrum of MOF 2 after hydrolysis of 11- 13 C (blue line). The isotopically labeled carbon atoms are lettered ( a – c ). c Hydrolisis of 11 with sodium methoxide to give chiral fragment 12 , and synthesis of 12 by enzymatic hydrolysis of diester 13 . Full size image With the above data in mind, the hydrolysis of brutieridin 11 was attempted with MOF 2 . A combined 1 H NMR, ultraviolet–visible spectrophotometry (UV–Vis), diffuse-reflectance UV–Vis spectrophotometry (DR–UV–Vis) and Fourier-transformed infrared spectroscopy (FT-IR) study was performed in order to follow concomitantly the fate of 11 in solution and within MOF 2 . 1 H NMR results (Supplementary Fig. 11 ) show that the hydrolysis indeed occurs. The alkyl fragment 11a progressively disappears from the solution, and the aromatic fragment transforms into a more symmetric aromatic molecule that persists in solution. This new aromatic molecule is the quinone fragment, according to UV–Vis and FT-IR (Supplementary Fig. 12 ) and also to GC-MS analysis (Supplementary Fig. 13 ), akin to what occurred during the hydrolysis of naringin 10 . DR–UV–Vis (Supplementary Fig. 14 ) and FT-IR measurements (Supplementary Fig. 15 ) of the solid MOF 2 after reaction reveal that the aromatic fragment does not incorporate into the pores, in line with the results observed for naringin 10 . To further confirm that the alkyl fragment 11a and not the aromatic part accommodates inside the MOF pores, 13 C isotopically labeled brutieridin ( 11– 13 C ) was prepared and hydrolyzed with MOF 2 (Supplementary Fig. 16 ). Figure 3b shows that only the methoxy signal (a) assignable to the methyl ester of 11a appears in the magic angle spinning (MAS) solid 13 C NMR spectrum of MOF 2 after hydrolysis of 11– 13 C . 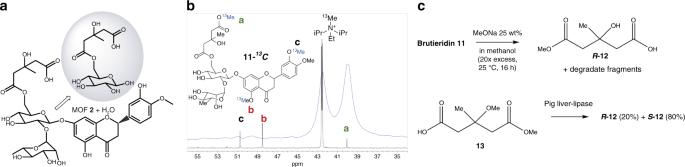Fig. 3: Hydrolysis of brutieridin 11. aChemical structure of brutieridin11. Gray-colored ellipse highlights the fragment11a, which contains the chiral carbon and encapsulates within the MOF after the break of the glycosidic bonds.bChemical structure and13C NMR spectrum of11-13Cin solution (black line), and MAS solid13C NMR spectrum of MOF2after hydrolysis of11-13C(blue line). The isotopically labeled carbon atoms are lettered (a–c).cHydrolisis of11with sodium methoxide to give chiral fragment12, and synthesis of12by enzymatic hydrolysis of diester13. The two anisolic signals (b and c) of the aromatic fragment, present in the 13 C NMR spectrum of 11– 13 C , are not present. These results strongly support the selective incorporation of the chiral alkyl fragment 11a to the crystalline MOF structure, yielding the novel hybrid material ( 11a )@{Ca II Cu II 6 [( S,S )-serimox] 3 (OH) 2 (H 2 O)}. 15H 2 O ( 11a@2 ), whose crystal structure as well as absolute configuration could now be elucidated by SCXRD analysis. Figure 4 shows the structure of 11a@2 , determined by SCXRD, which confirms the preservation of the networks of 2 after guests’ capture. 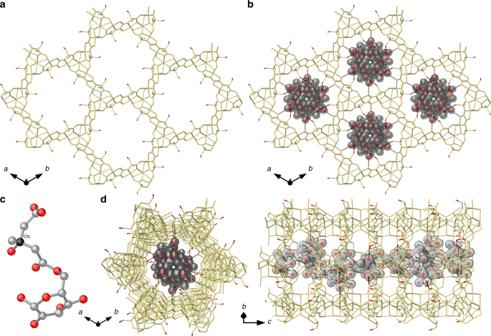Fig. 4: Crystal structure resolution of brutieridin 11. Views of the 3D open-framework of MOF2(a) and11a@2(b) along thec-axis (the crystallization water molecules are omitted for clarity). The 3D networks are depicted as gold sticks, with the only exception of serine residues oxygen atoms, which are represented as red sticks.cView of fragment of11aencapsulated within channels.dTop (left) and side (right) perspective views of a single channel of11a@2. Dashed lines represent hydrogen bonds between guest molecules involving also hydroxyl groups from the amino acid residue. The molecules of11aare shown as red (oxygen) and gray (carbon) stick/solid surfaces. 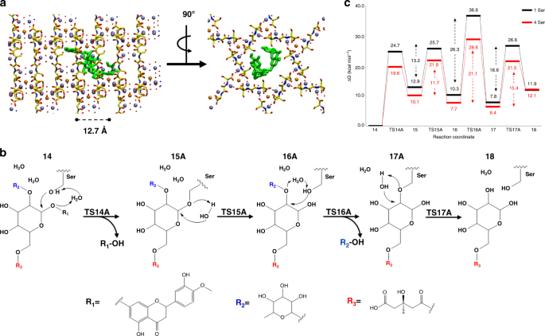Fig. 5: Theoretical mechanism for the MOF-catalyzed glycosyl hydrolysis. aThe best docked pose selected on the basis of the applied geometrical and energetic filters. The studied catalytic mechanisms (b) followed in the hydrolysis reaction of11by MOF2and related PES (c) calculated at B3LYP-D3/6-311 + G(2d,2p)|UFF//B3LYP/6-31G(d)|UFF level of theory. It is isomorphic to 2 crystallizing in the P 6 3 chiral space group of the hexagonal system and consists of a chiral honeycomb-like three-dimensional (3D) calcium(II)–copper(II) network, featuring functional hexagonal channels of ca. 0.9 nm as virtual diameter. The flexible hydroxyl (–OH) groups of the serine amino acid remain confined and stabilized by lattice water molecules, in the highly hydrophilic pores of the MOF (Fig. 4 and Supplementary Figs. 17 – 19 ). In these solvated nanospace, SCXRD underpinned 11a molecules disclosing their configurations and locations, despite the persistent disorder. The uni-nodal acs six-connected net is built up from trans oxamidato-bridged dicopper(II) units, {Cu II 2 [(S,S)-serimox]} (Fig. 4 ), which act as linkers between the Ca II ions through the carboxylate groups (Supplementary Fig. 1 ). Neighboring Cu 2+ and Cu 2+ /Ca 2+ ions are further interconnected by aqua/hydroxo groups (in a 1:2 statistical distribution) linked in a μ 3 fashion (Supplementary Fig. 1c ). Guest molecules of 11a reside in the pores, packed via hydrogen bonds interactions, mediated by serine derivative arms (Fig. 4b–d and Supplementary Figs. 17 – 19 ). Moreover, intermolecular interactions of the chiral net of MOF 2 enabled that the chiral carbon of the HMG side chain of 11a unveiled the R absolute configuration (Fig. 4c and Supplementary Fig. 20 ), with its bounded hydroxyl group directly interacting with methyl alcohol arm of the MOF (O5′···O1H ser = 3.014(10) Å). The detailed structures showed 11a arrangements (with a 1:3 statistical distribution, see Supplementary Methods for details and Supplementary Fig. 21 ), driven by the nature and size of the guest. In-depth analysis of the crystal structure reveals chiral 11a molecules packed via a plethora of strong H-bonds, as expected for a polar molecule (Fig. 4 and Supplementary Figs. 18 and 19 ), involving hydroxyl serine derivative arms directly linked to hydroxyl groups attached to both sugar moiety or HMG side chain [O···O distances varying in the range 2.73(1)–3.01(1) Å] (Supplementary Fig. 19 ). Oxamate oxygen atoms from the coordination network assist with strong hydrogen bonds involving carboxyl of HMG [O oxamate ···O carboxyl distances of 2.69(1) Å]. The vastly solvated nano-confined space further supports the host–guest recognition process, mediating the interaction with the net by lattice water molecules acting as bridge between host and guests to reach the serine derivative arms [shortest O 11A ···O W and related Ow···O ser distances of 2.94(1) and 2.68(1) Å, respectively], also involving the innate flexible carboxyl terminus of HMG side chain. This is reminiscent of the interaction mechanisms found in glycosidases enzymes [40] . Fig. 4: Crystal structure resolution of brutieridin 11. Views of the 3D open-framework of MOF 2 ( a ) and 11a@2 ( b ) along the c -axis (the crystallization water molecules are omitted for clarity). The 3D networks are depicted as gold sticks, with the only exception of serine residues oxygen atoms, which are represented as red sticks. c View of fragment of 11a encapsulated within channels. d Top (left) and side (right) perspective views of a single channel of 11a@2 . Dashed lines represent hydrogen bonds between guest molecules involving also hydroxyl groups from the amino acid residue. The molecules of 11a are shown as red (oxygen) and gray (carbon) stick/solid surfaces. Full size image Figure 3c shows that the controlled hydrolysis of brutieridin 11 with sodium methoxide gives the fragment derivative R - 12 by chiral-phase GC analysis, together with significant amounts of the epimerized fragment and some other degraded fragments of the natural product, as determined with an independently synthesized, enantiomerically enriched sample of 12 obtained after enzymatic hydrolysis of diester 13 with pig liver estearase. Thus, one can say that the R configuration is thus obtained within MOF 2 and also by conventional hydrolysis. This result strongly supports the validity of the crystallization method to give the correct absolute configuration of unknown products by SCXRD. Mechanism of the MOF-catalyzed glycosyl hydrolysis MOF 2 exposes, to outer molecules, a high number of densely packed alcohol groups, within a nanometer confined space, just as it occurs in the silanol nests of zeolites [8] , [9] . Thus, a particular acidification of adsorbed water, promoted by the cooperativeness between nearby methyl alcohols in MOF 2 , may occur. In order to discard potentially acidified water by interaction with the Cu II atoms of the MOF network, the building block Cu 2 II [(S,S)-serimox] was also tested as a catalyst for glycosyl hydrolysis in wet conditions, and the results showed a catalytic activity of the free Cu II species one order of magnitude lower than MOF 2 (Supplementary Fig. 22 ). Complementary, a filtration test showed that no leaching of active species occurs (Supplementary Fig. 23 ). Kinetic experiments with different amounts of reagents and catalyst (Supplementary Fig. 24 ) showed that the reaction orders for MOF 2 , ketal 4 , and water are 1, 1, and 0, respectively, thus giving a rate equation v 0 = k exp [ 2 ][ 4 ]. The role of adsorbed water was further examined by dehydrating MOF 2 at 80 °C under high vacuum (10 −4 mbar) during 16 h, and then performing the reaction with ketal 4 in anhydrous solvent, or adding 2 eq. of water to the reaction mixture at 60 °C. The results (Supplementary Fig. 25 ) show a 1/3 decrease of the hydrolysis rate compared to the original hydrated MOF 2 . These results support the catalytic action of water adsorbed in the alcohol network. Kinetic studies at different temperatures (25, 40, 60, and 80 °C) were carried out to calculate the activation energy of the glycolysis, which according to an Arrhenius plot was 15.0 kcal mol −1 . The catalysis should occur mainly inside the MOF pores rather than on its external surface, as supported by the easier reactivity of small molecules, the saturation of the solid material with the bigger molecules and the X-ray data of the encapsulated fragments. Computational studies were then performed to elucidate the possible mechanism of the glycosyl hydrolysis within MOF 2 (see Supplementary Methods ), and the results are shown in Fig. 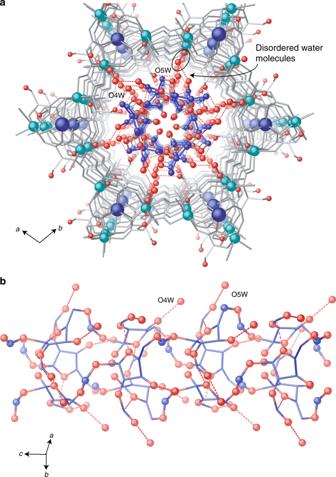5 . First, ten different complexes were generated by molecular recognition of 11 into the channel of MOF 2 (Supplementary Fig. 26 ). Fig. 2: Crystal structure of 1a@2. aPerspective view alongccrystallographic axis of a single channel underlining pores filled by guest molecules depicted as blue sticks with the only exception of oxygen atoms, depicted as red spheres. The H-bond interactions are depicted as red dashed lines. Disordered positions of lattice water molecules having a key role in host–guest interactions are highlighted (see details of refinement inSupplementary Methods).bSupramolecular chains of1amolecules packed in pores of2propagating along the direction of channels (all possible orientations are included). Carbon are represented by blue sticks whereas oxygen atoms of guest molecules and water molecules mediating host–guest interactions are represented by red spheres. Based on the applied geometrical and energetic filters (see Supplementary Table 2 ), which evidenced that all the examined poses share a common orientation inside the channel of MOF 2 , the best docked pose was isolated (Fig. 5a ) and used as starting structure in the Quantum Mechanics/Molecular Mechanics-Our own N-layered Integrated molecular Orbitals and Molecular mechanics (QM/MM–ONIOM) investigation (Supplementary Figs. 27 and 28 ). According to the calculations, the energetically favored mechanism for the hydrolysis of 11 within MOF 2 (see Fig. 5b, c ) occurs by sequential cleavage of the two acetal C–O bonds, to release first the aromatic (R1) and then the cyclic aliphatic (R2) moieties, through the formation of intermediates bound to the serine residues ( 15A and 17A in Fig. 5b ). The potential energy surface (PES) related to the mechanism of Fig. 5b , black line of Fig. 5c , evidences that the hydrolysis of R1 (TS14A, 24.7 kcal mol −1 ) and R2 (TS16A, 26.3 kcal mol −1 ) occurs with comparable barriers. The energy barriers associated with an alternative mechanism where R2 is released before R1 (Supplementary Fig. 29 ) and also in the absence of MOF 2 (Supplementary Fig. 30 ) are significantly higher in both cases. Moreover, the calculations also highlight that the increased number of serine moieties (four versus one, see red line of Fig. 5c ) leads to a lowering of the energy barriers (19.6 and 21.1 kcal mol −1 , for TS14A and TS16A, respectively). This supports the synergic effect of the alcohol arms in the hydrophilic nano-confined space of the MOF and, extrapolating to the higher number of serine moieties present within MOF 2 , nicely points to the experimental value (15.0 kcal mol −1 ) obtained for the hydrolysis activation energy. It must be noticed that glycosyl hydrolysis occurs in Nature by two different mechanisms, either in one-step with acid/base sites and inversion of chirality (inverting glycoside hydrolases) or in two different steps with acid/nucleophile sites and retention of the starting chirality (retaining glycoside hydrolases). The catalytic action of MOF 2 perfectly lies on the retaining type hydrolases, with the combined action of mild acid sites (water) and nucleophile sites (alcohols) in a confined space. Fig. 5: Theoretical mechanism for the MOF-catalyzed glycosyl hydrolysis. a The best docked pose selected on the basis of the applied geometrical and energetic filters. The studied catalytic mechanisms ( b ) followed in the hydrolysis reaction of 11 by MOF 2 and related PES ( c ) calculated at B3LYP-D3/6-311 + G(2d,2p)|UFF//B3LYP/6-31G(d)|UFF level of theory. Full size image An amino acid-derived MOF ( 2 ), densely decorated with methyl alcohol arms, is not only capable to hydrolyze glycosyl bonds like retaining hydrolase enzymes, without the participation of formal protons, but also to act as a vessel encapsulating the released chiral fragment and allowing the absolute structural determination of the natural product by SCXRD. The present results constitute a clear step forward on the use of MOFs in enzymatic catalysis [41] , [42] , where commonly their catalytic activity arises from preformed encapsulated active species. Also, let us anticipate that this bioinspired methodology with MOFs [41] , [43] , [44] , [45] , [46] , [47] could have future application in the MOF-driven structural characterization [48] , [49] of more natural product structures [15] , [50] , [51] . Preparation of 1a@2 Well-formed hexagonal green prisms of 1a@2 (( 1a )@{Ca II Cu II 6 [( S,S )-serimox] 3 (OH) 2 (H 2 O)}. 19H 2 O, where 1a = 1,3,4,6-Tetra- O -acetylfructofuranoside), which were suitable for X-ray diffraction, were obtained by soaking crystals of 2 (ca. 5.0 mg) in saturated water solutions of sucrose octaacetate ( 1 ), for 48 h at temperature of 50 °C. The crystals were isolated by filtration on paper and air-dried. 1a@2: Anal. : calcd for C 38 Cu 6 CaH 82 N 6 O 56 (1940.42): C, 23.52; H, 4.26; N, 4.33%. Found: C, 23.50; H, 4.21; N, 4.36%. IR (KBr): ν = 1625, 1611, 1610 cm −1 (C=O). Preparation of 11a@2 Well-shaped hexagonal prisms of 11a@2 (( 11a )@{Ca II Cu II 6 [( S,S )-serimox] 3 (OH) 2 (H 2 O)}. 15H 2 O, where 11a = 6- O -(3′–hydroxy-3′-methylglutaryl)-glucopyranose)), suitable for SCXRD, could be obtained by soaking crystals of 2 (which had been treated before through a solvent exchange process for a week, recharging fresh acetonitrile solvent daily) in a saturated acetonitrile solution containing hesperetin 7-(2′′-R-rhamnosyl-6′′-(3′′′′-hydroxy-3′′′′-methylglutaryl)-glucoside) (brutieridin 11 ) during two weeks. After this period, crystals were isolated by filtration and air-dried. Anal. : calcd for C 36 Cu 6 CaH 74 N 6 O 52 (1844.33): C, 23.44; H, 4.04; N, 4.56%. Found: C, 23.39; H, 4.01; N, 4.57%; IR (KBr): ν = 1637, 1613, 1608 cm −1 (C – O). Catalytic procedures MOF 2 or MOF 3 (37.5 mg, 100 wt%) were placed in a 2 ml vial equipped with a magnetic stir bar, and the corresponding amount of CD 3 CN (0.75 ml) was added. Then, the corresponding amount of naringin 10 (37.5 mg) was added at room temperature. The mixture was sealed and magnetically stirred in a pre-heated oil bath at 60 °C. For kinetic experiments, individual reactions were placed for each point and after centrifugation, the supernatant of the mixture reaction was periodically taken and analyzed by NMR. The same procedure was followed for brutieridin 11 . Preparation of 13 C isotopically labeled 11– 13 C Brutieridin 11 (10 mg 0.013 mmol) was placed in a round-bottomed flask equipped with a magnetic stir bar, and CD 3 CN (2 ml). Then, N , N -Diisopropylethylamine (7 μl, 0.039 mmol) and 13 CH 3 I (5 μl, 0.078 mmol) were added via syringe at 0 °C. The mixture was sealed and magnetically stirred at room temperature for 12 h. After that, the reaction mixture was analyzed by 13 C NMR. Single-crystal X-ray diffraction Crystal data for 1a@2 and 11a@2 : Hexagonal, space group P 6 3 , T = 90(2) K, Z = 2; 1a@2 : C 38 Cu 6 CaH 82 N 6 O 56 , a = 17.7840(16) Å, c = 12.5090(14) Å, V = 3426.2(7) Å 3 , σ = 1.881 g cm 3 , µ (mm −1 ) = 2.031; Absolute structure parameter (Flack) of 0.12(2). 11a@2 : C 36 Cu 6 CaH 74 N 6 O 52 , a = 17.9667(15) Å, c = 12.6886(12) Å, V = 3547.2(7) Å 3 , σ =  1.727 g cm 3 , µ (mm −1 ) = 1.953. Absolute structure parameter (Flack) of 0.13(2). Further details can be found in the Supplementary Information . Computational details The solved X-ray structure of MOF 2 has been adopted as starting point in the computational investigation. The molecular recognition has been applied to dock substrate 11 into MOF 2 , generating ten different poses. The best docked pose has been undertaken to QMMM investigations. The same computational protocol has been previously applied in recent works. Further detailed description of the used methods is given in Supplementary Methods .